Atomically precise interfaces from non-stoichiometric deposition Complex oxide heterostructures display some of the most chemically abrupt, atomically precise interfaces, which is advantageous when constructing new interface phases with emergent properties by juxtaposing incompatible ground states. One might assume that atomically precise interfaces result from stoichiometric growth. Here we show that the most precise control is, however, obtained by using deliberate and specific non-stoichiometric growth conditions. For the precise growth of Sr n +1 Ti n O n +1 Ruddlesden–Popper (RP) phases, stoichiometric deposition leads to the loss of the first RP rock-salt double layer, but growing with a strontium-rich surface layer restores the bulk stoichiometry and ordering of the subsurface RP structure. Our results dramatically expand the materials that can be prepared in epitaxial heterostructures with precise interface control—from just the n =∞ end members (perovskites) to the entire RP homologous series—enabling the exploration of novel quantum phenomena at a richer variety of oxide interfaces. Members of the Ruddlesden–Popper (RP) homologous series [1] , [2] , [3] ( Supplementary Fig. 1 ) include high temperature superconductors [4] , colossal-magnetoresistance oxides [5] and systems that, with changing dimensionality, are controlled by n , vary from spin-triplet superconductors [6] , [7] to unconventional ferromagnets [8] , [9] . Just as the ability to precisely engineer interfaces between perovskites (the n =∞ end member of the RP series) has led to emergent properties at perovskite interfaces, including metal-insulator transitions [10] , [11] , high electron mobility [12] , large negative magnetoresistance [13] and superconductivity [14] , [15] , the dimensionality reduction, point defect accommodation [16] and additional novel properties offered by RP phases provide exciting opportunities for oxide interfaces, provided they can be prepared with atomic precision. Limited by thermodynamic stability, RP materials with 3< n <∞ cannot be synthesized by conventional solid state techniques [1] , [2] , [17] , [18] or codeposition thin film growth techniques [19] , [20] , [21] , [22] , [23] , [24] , [25] , [26] , [27] , [28] , [29] , [30] . The ‘layer-by-layer’ method, in which the constituent species are supplied sequentially following the exact order of monolayers in the growth direction of the targeted structure, has been employed by both pulsed-laser deposition [31] , [32] , [33] and reactive molecular-beam epitaxy (MBE) [34] , [35] , [36] , to yield well-ordered single-phase epitaxial films of Sr n +1 Ti n O 3 n +1 (refs 37 , 38 ), Sr n +1 Ru n O 3 n +1 (ref. 39 ) and Ca n +1 Mn n O 3 n +1 (ref. 40 ) RP phases with n as high as 10 (ref. 41 ). This ability recently led to a breakthrough in tunable microwave dielectric materials [42] . In addition to being able to achieve RP phases with intermediate values of n , this shuttered method involves significantly lower growth temperatures, compared with the codeposition method. Although sequentially supplying monolayer doses of the constituent species does affect growth in a way that yields the desired layering [35] , [37] , [38] , [39] , [40] , [42] , [43] , the microscopic details of how the supplied composition modulation affects growth, and more specifically the growth mechanism of RP phases, remains a mystery. This frequently limits the precise control of the interfaces and thus the investigation of oxide interfaces based on RP materials. Here we study the growth mechanism and interface engineering of RP titanate films using a combination of MBE, in situ reflection high-energy electron diffraction (RHEED), angle-dependent X-ray photoemission spectroscopy (XPS), high-resolution scanning transmission electron microscopy (STEM) and first-principles simulations based on density functional theory (DFT). We obtain high crystalline quality RP films using the normal ‘layer-by-layer’ growth process in which the constituent species are supplied sequentially following the ‘layer-by-layer’ order of monolayers in the growth direction of the targeted structure. Interestingly, we observe an unexpected interface between RP films and a substrate with known termination in which the first SrO–SrO rock-salt double layer (SrO double layer) is always missing using this normal ‘layer-by-layer’ growth technique. Further, the surface composition, including those designed to be terminated with TiO 2 , remains SrO. This can be understood as a natural consequence of the presence of an additional SrO monolayer that rides the surface during the growth of SrO double layers. We then develop an optimized non-stoichiometric growth process and obtain the desired atomically sharp interface through ‘layer-by-layer’ engineering. Our work expands the material systems that can be engineered with atomic-layer precision from the n =∞ end member ( AB O 3 perovskites) to encompass the entire RP family, and thus greatly expands the variety of oxide interfaces that can be prepared to investigate novel quantum phenomena. Missing initial SrO double layer The shuttered ‘layer-by-layer’ growth method using MBE is schematically shown in Fig. 1a . During the growth, the fluxes from elemental strontium and titanium sources are shuttered alternately with accurate timing control to provide precise deposition of SrO and TiO 2 monolayers onto the (110) DyScO 3 substrate in the desired sequence. The oxidant (O 2 +10% O 3 ) is supplied during the whole growth and cooling process to minimize the formation of oxygen vacancies. In situ RHEED is employed to monitor the surface evolution during growth and the intensity oscillations of RHEED streaks are used to provide accurate shutter timing calibrations [44] . The thicknesses of all RP films grown on DyScO 3 are ~500 Å. X-ray diffraction (XRD) measurements show intense and narrow peaks and clear thickness (Kiessig) fringes at the expected locations of phase-pure Sr n +1 Ti n O 3 n +1 with n =2, 3, 4 and 6 ( Fig. 1b ). The thickness fringes are more clearly shown in a zoomed-in plot ( Supplementary Fig. 2 ). Atomic-resolution STEM images confirm the structures consist of n perovskite layers separated by SrO double layers. Surprisingly, all samples are missing the initial SrO double layer ( Fig. 1c–f ), showing that the simple ‘layer-by-layer’ deposition cartoon ( Fig. 1a ) is incorrect. Away from the substrate interface, the SrO double layers are still present, consistent with the XRD results. The missing initial SrO double layer cannot be explained as simply being due to an imperfect flux calibration. A small deviation (1%) in the fluxes will lead to clear peak splitting and position shifts in the XRD pattern [37] , [39] , [42] , inconsistent with our XRD data. Moreover, the microscopic structure of RP titanates has been shown to be very sensitive to its stoichiometry [45] . The RP films, other than the n =4 one, show very few vertical faults, but all are missing the first SrO double layer, implying this is not simply because of an imperfect calibration of the monolayer doses supplied to the substrate. Furthermore, it is not related to the surface termination of the substrates. The scandate substrates were prepared to be terminated with ScO 2 (ref. 46 ). As the initial deposited layer is SrO, a partial extra SrO layer would be expected if the substrate surface were not perfectly terminated with ScO 2 , inconsistent with the observation of the missing SrO double layer in our case. 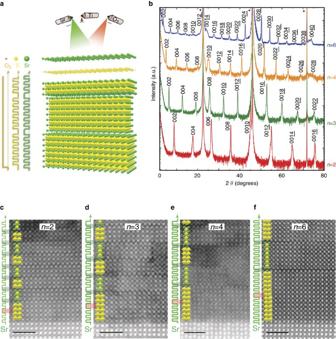Figure 1: The missing initial SrO double layer near the interface of all RP films. (a) A spray painting cartoon illustrating the ‘layer-by-layer’ MBE growth idealization of ann=6 RP film. The shutter sequence diagrams for Sr, Ti and O3fluxes are shown on the left. (b)θ−2θX-ray diffraction of RP films withn=2, 3, 4 and 6 grown on (110) DyScO3substrates. Substrate peaks are labelled with an * and the plots are offset for clarity. (c–f) ADF-STEM images from corresponding RP films, showing an unexpected absence of the initial SrO double layer near the substrate interface of all RP films. The atomic structure model and Sr-flux shutter timing diagram of each film are shown on the left. The positions of present and absent SrO double layers are highlighted in green and red, respectively. Then=4 film shows imperfect growth with some vertical faults and lower contrast between theA-site andB-site atoms in some regions due to averaging over two grains in the beam direction. The image of then=6 RP film was taken on an aberration-corrected Nion UltraSTEM, and thus has higher resolution compared to the other images. Scale bars, 2 nm. Figure 1: The missing initial SrO double layer near the interface of all RP films. ( a ) A spray painting cartoon illustrating the ‘layer-by-layer’ MBE growth idealization of an n =6 RP film. The shutter sequence diagrams for Sr, Ti and O 3 fluxes are shown on the left. ( b ) θ −2 θ X-ray diffraction of RP films with n =2, 3, 4 and 6 grown on (110) DyScO 3 substrates. Substrate peaks are labelled with an * and the plots are offset for clarity. ( c – f ) ADF-STEM images from corresponding RP films, showing an unexpected absence of the initial SrO double layer near the substrate interface of all RP films. The atomic structure model and Sr-flux shutter timing diagram of each film are shown on the left. The positions of present and absent SrO double layers are highlighted in green and red, respectively. The n =4 film shows imperfect growth with some vertical faults and lower contrast between the A -site and B -site atoms in some regions due to averaging over two grains in the beam direction. The image of the n =6 RP film was taken on an aberration-corrected Nion UltraSTEM, and thus has higher resolution compared to the other images. Scale bars, 2 nm. Full size image SrO-terminated surface of RP films Moreover, we observe an unexpected SrO-terminated surface of all RP titanate films, including those designed to be terminated with TiO 2 . To study the surface termination, we performed angle-dependent XPS measurements on n =1 RP films ( Fig. 2 ); the results are representative of RP titanate films containing SrO double layers, that is, RPs with finite n . Two Sr 2 TiO 4 films were grown on TiO 2 -terminated (001) SrTiO 3 substrates using the shuttered ‘layer-by-layer’ growth method and their final deposited layers were designed to be SrO and TiO 2 , respectively. For comparison, we also grew Sr 2 TiO 4 films using the co-deposition method, where the shutters of all constituent elemental sources were kept open simultaneously during the entire growth process. As the SrTiO 3 substrates we used were terminated with TiO 2 (ref. 47 ), the co-deposition method would be expected to yield a TiO 2 termination of the film. The structural perfection of the films were characterized by XRD measurements ( Supplementary Fig. 3 ). 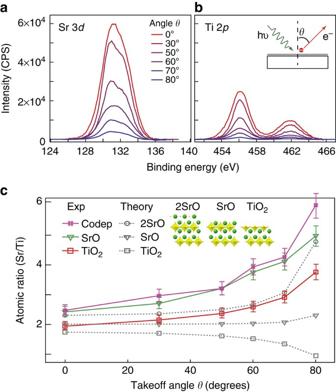Figure 2: SrO-terminated surface of RP films studied by angle-dependent XPS. Angle-dependent XPS spectra of (a) Sr 3dand (b) Ti 2ppeaks of Sr2TiO4films. Inset: schematic of the XPS apparatus. (c) Angle-dependent Sr/Ti atomic ratio together with simulations, indicating that the surface is terminated with one or more monolayers of SrO for all RP films. The simulations are theoretical estimations of the Sr/Ti atomic ratio made using equation (1) in the Methods section. Figure 2: SrO-terminated surface of RP films studied by angle-dependent XPS. Angle-dependent XPS spectra of ( a ) Sr 3 d and ( b ) Ti 2 p peaks of Sr 2 TiO 4 films. Inset: schematic of the XPS apparatus. ( c ) Angle-dependent Sr/Ti atomic ratio together with simulations, indicating that the surface is terminated with one or more monolayers of SrO for all RP films. The simulations are theoretical estimations of the Sr/Ti atomic ratio made using equation (1) in the Methods section. Full size image In Fig. 2a,b , the XPS profile of Sr 3 d and Ti 2 p peaks shows a clear dependence on the takeoff angle. The area of each peak is calculated after subtracting a Shirley background [48] (not shown) and is used to determine the atomic concentration for that element after being scaled by a relative sensitivity factor. The extracted atomic Sr/Ti ratio clearly increases with takeoff angle θ for all films ( Fig. 2c ). In angle-dependent XPS, the photoelectron yield decreases exponentially with sampling depth at a fixed takeoff angle. The total intensity of photoelectrons is a weighted sum of the signals emanating from all sampling depths (see Methods section). As the takeoff angle increases, the total intensity of photoelectrons is more surface sensitive. Comparison with the theoretical simulations (dashed lines) implies that all films are terminated with one or more SrO layers. The clear angular dependence of the atomic Sr/Ti ratio unambiguously implies an SrO-terminated surface for all of the Sr 2 TiO 4 films, even those attempted to be TiO 2 terminated. Microscopic growth mechanism of SrO double layers To reconcile these unexpected observations of a missing interfacial SrO double layer and the ever-present SrO-terminated surface, we investigate the microscopic growth mechanism of RP films, more specifically the SrO double layer, by studying the growth of a single SrO double layer in thick SrTiO 3 films. To avoid strain effects and the introduction of defects from relaxation, we used (001) (LaAlO 3 ) 0.29 (SrAl 0.5 Ta 0.5 O 3 ) 0.71 (LSAT) substrates, as they are well lattice matched with RP titanates with low n . After growth, a 10-nm-thick amorphous La 2 O 3 capping layer was deposited on the film surface at room temperature to protect the surface for high-resolution STEM measurements. We first grew a 10 unit cell (u.c.) thick (001) SrTiO 3 film on (001) LSAT to verify the growth conditions. Indeed, the STEM image shows the SrTiO 3 to have the expected 10 u.c. thickness by counting the number of SrO layers ( Fig. 3a ). For the second sample, we attempted to insert an SrO double layer into the middle of the 10-u.c.-thick SrTiO 3 structure by depositing one extra SrO layer after the first 5 u.c. of SrTiO 3 . Surprisingly, the final structure shows no trace of an SrO double layer at any location ( Fig. 3b ). Instead, we find an extra SrO layer on the top surface of the film, suggesting the inserted extra SrO layer switches position with the following TiO 2 layer as schematically shown in the cartoon model ( Fig. 3d ). This position switching process continues until the end of the film growth, resulting in an extra SrO monolayer on the top surface. 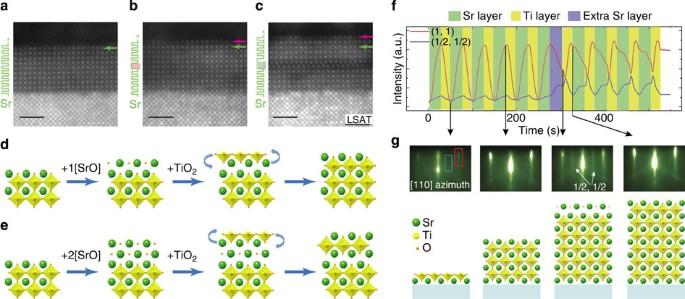Figure 3: Microscopic growth mechanism of SrO double layers. ADF-STEM images from 10-u.c.-thick (001) SrTiO3films grown on (001) LSAT substrates with an attempt to insert (a) no, (b) 1 and (c) 2 extra SrO layers halfway through the growth of the 10-u.c.-thick SrTiO3film. An SrO double layer is formed in the last case only. The excess SrO layer is observed on the film surface, which is indicated by the magenta arrow. The green arrows indicate the tenth SrO layer. Scale bars, 2 nm. Cartoon models showing the SrO–TiO2switching mechanism in forming the (d) missing and (e) incorporating SrO double layer. (f) Shuttered RHEED intensity oscillations of (1, 1) and (1/2, 1/2) diffraction streaks within the light red and light blue boxes, respectively, during the growth of the artificial structure inb, showing the evolution of the surface diffraction pattern along the [110] azimuth of SrTiO3. (g) RHEED patterns along the [110] SrTiO3azimuth and corresponding cartoon models taken at different stages of growth indicated by the arrows. Figure 3: Microscopic growth mechanism of SrO double layers. ADF-STEM images from 10-u.c.-thick (001) SrTiO 3 films grown on (001) LSAT substrates with an attempt to insert ( a ) no, ( b ) 1 and ( c ) 2 extra SrO layers halfway through the growth of the 10-u.c.-thick SrTiO 3 film. An SrO double layer is formed in the last case only. The excess SrO layer is observed on the film surface, which is indicated by the magenta arrow. The green arrows indicate the tenth SrO layer. Scale bars, 2 nm. Cartoon models showing the SrO–TiO 2 switching mechanism in forming the ( d ) missing and ( e ) incorporating SrO double layer. ( f ) Shuttered RHEED intensity oscillations of (1, 1) and (1/2, 1/2) diffraction streaks within the light red and light blue boxes, respectively, during the growth of the artificial structure in b , showing the evolution of the surface diffraction pattern along the [110] azimuth of SrTiO 3 . ( g ) RHEED patterns along the [110] SrTiO 3 azimuth and corresponding cartoon models taken at different stages of growth indicated by the arrows. Full size image This hypothesis is further supported by our real-time in situ RHEED measurements ( Fig. 3f,g ). RHEED patterns are very surface sensitive, and the maximum and minimum intensity of the (1,1) diffraction streak correspond to the SrO-terminated and TiO 2 -terminated surfaces of SrTiO 3 , respectively [44] . One period of the observed shuttered intensity oscillation corresponds to the growth of a full u.c. of SrTiO 3 . In contrast, the presence of half-integer RHEED streaks at positions along the [110] azimuth of (001) SrTiO 3 indicate excess SrO (more than one full layer) on the surface [49] , [50] , [51] . In Fig. 3f , the shuttered RHEED intensity oscillation shows a significant increase of the (1/2, 1/2) peak during the deposition of the extra SrO layer, suggesting an increase of excess SrO on the surface of the film. After depositing the following TiO 2 layer, however, the intensity of (1/2, 1/2) streaks decreases to a minimum, while the intensity of (1, 1) streaks goes back to a maximum value, identical to the SrO-terminated surface in a perfect SrTiO 3 structure. The corresponding RHEED pattern is also identical to the SrO-terminated surface, implying the SrO layer indeed switched position with the TiO 2 layer. During the growth of the last 5 u.c. of SrTiO 3 of this second sample, the intensity of the (1/2, 1/2) and (1,1) peaks oscillate periodically in an anti-phase manner, suggesting that such an SrO-TiO 2 switching process continues to take place until the end of growth, leaving an SrO-terminated surface. This is consistent with our STEM measurements and also with recent in situ synchrotron x-ray scattering measurements during the growth of Sr 2 TiO 4 , La 2 NiO 4 , and La 3 Ni 2 O 7 (ref. 52 ). This behaviour can also be understood from energy considerations. In RP structures with low n , the distance between SrO and TiO 2 layers is 1.92 Å, while the distance between two SrO layers is 2.56 Å (ref. 53 ), which generally would imply a weaker bond energy between two such rock-salt planes. This is a common feature of all RP materials. As a consequence, the natural cleavage plane of RP phases, such as layered manganites [54] and ruthenates [55] , is between the rock-salt double layers. Thus, we expect a TiO 2 layer deposited on top of an SrO double layer to find a lower energy configuration by switching positions with the uppermost SrO layer and residing between them where it can bond with both SrO layers. Indeed, our DFT calculations support this qualitative notion and show that the structures after switching of TiO 2 and SrO layers are energetically more favourable than before the switching ( Fig. 4 ). Four different types of free surfaces have been simulated using periodic symmetrically terminated slabs, schematically shown in Fig. 4a–d . Two of them ( Fig. 4a,b ) contain 9 layers of SrO and 8 layers of TiO 2 , while the other two ( Fig. 4c,d ) contain 11 layers of SrO and 8 layers of TiO 2 . For each pair of structures with the same overall stoichiometry, the first TiO 2 layer has been placed in different positions, corresponding to the possible diffusion of titanium into the underlying structure: (i) at the top most atomic layer with two ( Fig. 4a ) or three ( Fig. 4c ) consecutive layers of SrO beneath it ( Fig. 4a,c ) and (ii) at the subsurface layer, in between two SrO planes ( Fig. 4b,d ). The vacuum regions were thicker than 12 Å (more than 3 u.c. of SrTiO 3 ), large enough to avoid interactions between periodic replicas. Symmetric slabs were used to only focus on the effects of the surfaces. The in-plane lattice constants were chosen to match the theoretical lattice constant of bulk SrTiO 3 (3.874 Å) (ref. 56 ). The out-of-plane lattice constants were free to relax together with the atomic positions until the value of the maximum component of the force on any atom fell below 10 meV Å −1 . 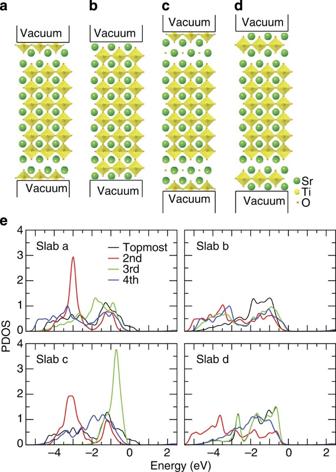Figure 4: Unfavourable TiO2-terminated surface from DFT calculations. (a–d) Schematic diagram of the slabs considered, having various terminations. (e) Partial density of states projected onto the O 2porbitals of the topmost four layers from the surface inward. The zero energy level is the top of the valence band computed from the position of the local band edge at the central SrO layer in each slab. The Fermi energy always lies within the gap. Figure 4: Unfavourable TiO 2 -terminated surface from DFT calculations. ( a – d ) Schematic diagram of the slabs considered, having various terminations. ( e ) Partial density of states projected onto the O 2 p orbitals of the topmost four layers from the surface inward. The zero energy level is the top of the valence band computed from the position of the local band edge at the central SrO layer in each slab. The Fermi energy always lies within the gap. Full size image The calculated total free energy differences (Δ E ) are 0.76 eV between slab (a) and (b), and 1.20 eV between slab (c) and (d), implying a large energy gain by surrounding TiO 2 with SrO layers on both sides. These energetic considerations support the experimental observation about the tendency of the TiO 2 layers to diffuse down in between SrO layers. We also performed additional calculations to investigate whether the TiO 2 layer would penetrate more than one SrO layer when three consecutive SrO layers are present and form an SrO-SrO-TiO 2 -SrO... configuration. The calculations show that the total free energy of this configuration is higher (less stable) than the configuration in case (d) by 0.43 eV, in good agreement with the experimental observations (the TiO 2 layer only penetrates one SrO layer). Furthermore, beyond the energy of the different configurations, the energy barrier that the TiO 2 layer needs to overcome would probably increase when penetrating deeper, as the titanium atoms are now bonded with more atoms in all three dimensions, making the mechanism less realistic. These theoretical results can be understood from the evolution of the character of the bonding with the position of the TiO 2 layer in the different structures. In Fig. 4e , we plot the layer-by-layer projected density of states (PDOS) on an oxygen atom located in one of the four topmost layers. Slabs (a) and (c), with TiO 2 planes at the interface with vacuum, display states with energies just above the top of the bulk valence band with nearly pure O 2 p character (without hybridization with Ti 3 d levels). In fact, at the top of the bulk valence band, all of the O 2 p orbitals are hybridized to some extent with Ti 3 d states, which lowers the energy of the O 2 p orbitals. At the TiO 2 -terminated surface, the local symmetry and the crystal field splitting on the titanium atoms is different from bulk, together with their interaction with the oxygen atoms; as a consequence, the mixing of the states that shift the position of the valence bands as in the bulk case is no longer possible. Therefore, some of the O 2 p states remain close to the free-atom energy levels, intruding into the lower part of the gap. On the other hand, when the surface is SrO-terminated, every surface oxygen atom has a titanium atom below it with which it hybridizes, resulting in a lowering of the PDOS towards higher binding energies. In addition, when the topmost TiO 2 layer is surrounded by two SrO layers, as occurs in slabs (b) and (d), the PDOS on the nearest SrO planes more closely resembles that of the SrO planes in bulk SrTiO 3 than that of bulk SrO. This translates into a wider shape of the PDOS, spreading over higher binding energies. As a consequence of the partial covalent bonding in the perovskite, the sharp peaks located around 3.0 eV (slab (a)), and 0.7 and 3.0 eV (slab (c)) below the top of the valence band, which signify the strong ionic bonding in SrO, are distributed over larger energy windows in slab (b) and (d), respectively. Clearly, the energy of the TiO 2 plane will be lowered if it is not at the surface. Experimentally, the actual structures may have various types of defects and surface reconstructions. We should also point out that our simulations do not address the dynamical problem of the diffusion. Nonetheless, our calculations indicate that a TiO 2 -terminated surface atop more than one SrO layer is unstable with respect to inward migration and agree qualitatively with our experimental observations. This monolayer switching process is able to occur at the relatively high growth temperature utilized. Presumably, it could be kinetically avoided at sufficiently low growth temperature, but we have not investigated such conditions. Atomically precise interface control To obtain the desired control over where the SrO double-layer interfaces occur with atomic specificity, we grew a third sample into which two extra SrO layers were inserted into the middle of a 10-u.c.-thick SrTiO 3 structure. As shown in Fig. 3c , an SrO double layer appears at this location and an extra SrO layer is found on the surface. This suggests that the TiO 2 layer deposited subsequently to the extra two SrO layers only switched position with the top most SrO layer, leaving an SrO double layer ( Fig. 3e ) as shown in STEM measurements ( Fig. 3c ). This is again supported by an energy consideration in our DFT calculations. Guided by this cation switching model, we established an optimized growth recipe for RP titanate films by depositing one extra SrO layer at the substrate interface to form the one-SrO-monolayer-rich condition necessary for the controlled growth of subsequent SrO double layers at desired positions with atomic-layer specificity. In Fig. 5 , an n =6 RP film grown by this optimized non-stoichiometric deposition process indeed shows the desired interface. We also confirmed this optimized growth method on RP films with different n values as shown in Supplementary Fig. 4 ( n =5). 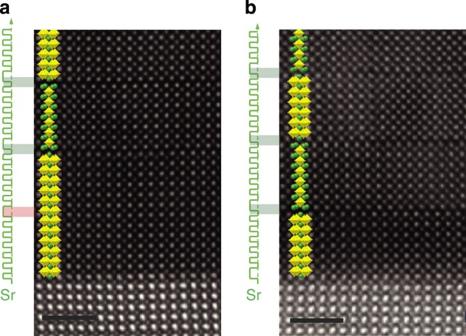Figure 5: Achievement of the desired interface inn=6 RP films through ‘layer-by-layer’ engineering. ADF-STEM images fromn=6 RP films grown on (110) DyScO3using (a) conventional and (b) revised shutter sequences, showing the successful growth of the targeted interface in the latter non-stoichiometric case. The positions of present and absent SrO double layers are highlighted in light blue and light red, respectively. Scale bars, 2 nm. Figure 5: Achievement of the desired interface in n =6 RP films through ‘layer-by-layer’ engineering. ADF-STEM images from n =6 RP films grown on (110) DyScO 3 using ( a ) conventional and ( b ) revised shutter sequences, showing the successful growth of the targeted interface in the latter non-stoichiometric case. The positions of present and absent SrO double layers are highlighted in light blue and light red, respectively. Scale bars, 2 nm. Full size image Through a series of experiments and calculations, we have elucidated the microscopic growth mechanism of SrO double layers in RP phases, which explains observations counter to the cartoon ‘layer-by-layer’ growth model ( Fig. 1a ). It has long been assumed that RP phases grow in the same layer-by-layer order that their constituent monolayers are deposited, but our results show this is untrue. We further show that a desired SrO double layer can be inserted with atomic layer precision into RP titanates through an optimized growth process. This demonstrates the power of non-stoichiometric deposition through ‘layer-by-layer’ engineering in growing atomically sharp interfaces at desired locations in complex oxide heterostructures. Our work provides a route to study novel interfacial phases containing any desired n member within the RP series. Reactive MBE film growth Sr n +1 Ti n O 3 n +1 RP titanate films with n up to six were deposited at a substrate temperature of 750–780 °C and an oxidant background pressure (O 2 + ~10% O 3 ) of 3 × 10 −7 −5 × 10 −7 Torr using Veeco 930 and Gen 10 oxide MBE systems. A low-temperature effusion cell and a Ti-Ball [57] were used to generate strontium and titanium molecular beams, respectively. A shuttered ‘layer-by-layer’ method was used to grow all samples in this work. The fluxes of strontium and titanium were initially calibrated using a quartz crystal microbalance and the precise monolayer shutter timing of the strontium and titanium doses were subsequently refined using RHEED intensity oscillations [44] . Scanning transmission electron microscopy Samples for STEM measurements were prepared by mechanical wedge polishing followed by short-time Ar-ion milling [58] . High-angle annular-dark-field STEM images were taken both on a 200-kV FEI Tecnai F20 SuperTWIN and on a 100-kV Nion UltraSTEM equipped with an aberration corrector [59] . STEM images, except the one shown in Fig. 1e ( n =4), were averaged over a few frames (pre-aligned using a cross-correlation algorithm) to reduce scan distortions. X-ray photoemission spectroscopy The ex situ angle-dependent XPS measurements were performed under ultrahigh-vacuum using monochromatic Al K α X-ray radiation. Samples were stored under ultra-high vacuum before XPS measurements to minimize the exposure of the samples to air. To prevent surface charging during the XPS measurements, the samples were irradiated with low-energy electrons. In angle-dependent XPS, the photoelectron yield decreases exponentially with sampling depth at a fixed takeoff angle. The total intensity for photoelectrons I j ( θ ), is a weighted sum of the signals emanating from all sampling depths [60] . where K j is a constant related to the elemental sensitivity and instrumental factors of atom j , n j,i represents the atom fraction composition of element j in the i th layer, Z i is the depth of the i th layer from the surface, λ j is the characteristic attenuation length for the photoelectrons originating from element j and θ is the takeoff angle of emission measured from the sample normal. The characteristic attenuation length λ j for the photoelectrons originating from Sr 3 d and Ti 2 p are calculated to be 25.69 and 20.77 Å, respectively, using the NIST Electron Effective-Attenuation-Length database [61] . The instrument-dependent constant K j can be cancelled out in calculating the atomic concentrations and ratios [60] . DFT calculations DFT calculations, in the local density approximation, were performed within a numerical atomic orbital method, as implemented in the Siesta code [62] . Core electrons were replaced by fully separable norm-conserving pseudopotentials. Because the large overlap between the semicore and valence states, the 3 s and 3 p electrons of titanium, and 4 s and 4 p electrons of strontium were considered as valence electrons and explicitly included in the simulations. The one-electron Kohn–Sham eigenvalues were expanded in a basis of strictly localized numerical atomic orbitals. We used a single-zeta basis set for the semicore states of titanium and strontium, and a double-zeta plus polarization for the valence states of all the atoms. For strontium, an extra shell of 4 d orbitals was added. Further details on the pseudopotentials and basis sets can be found in ref. 56 . The electronic density, Hartree and exchange-correlation potentials, as well as the corresponding matrix elements between the basis orbitals, were computed on a uniform real space grid with an equivalent plane-wave cutoff of 1,200 Ry in the representation of the charge density. A 12 × 12 × 1 Monkhorst–Pack mesh was used for the sampling of reciprocal space. To compute the PDOS, a non-self-consistent calculation within a grid of 60 × 60 × 2 was employed. To optimize the geometry of the structure, the out-of-plane lattice constants and the atomic positions were relaxed until the value of the maximum component of the force on any atom fell below 10 meV Å −1 . How to cite this article: Nie, Y. F. et al. Atomically precise interfaces from non-stoichiometric deposition. Nat. Commun. 5:4530 doi: 10.1038/ncomms5530 (2014).